The β-hydroxybutyrate receptor HCA2activates a neuroprotective subset of macrophages The ketone body β-hydroxybutyrate (BHB) is an endogenous factor protecting against stroke and neurodegenerative diseases, but its mode of action is unclear. Here we show in a stroke model that the hydroxy-carboxylic acid receptor 2 (HCA 2 , GPR109A) is required for the neuroprotective effect of BHB and a ketogenic diet, as this effect is lost in Hca 2 −/− mice. We further demonstrate that nicotinic acid, a clinically used HCA 2 agonist, reduces infarct size via a HCA 2 -mediated mechanism, and that noninflammatory Ly-6C Lo monocytes and/or macrophages infiltrating the ischemic brain also express HCA 2 . Using cell ablation and chimeric mice, we demonstrate that HCA 2 on monocytes and/or macrophages is required for the protective effect of nicotinic acid. The activation of HCA 2 induces a neuroprotective phenotype of monocytes and/or macrophages that depends on PGD 2 production by COX1 and the haematopoietic PGD 2 synthase. Our data suggest that HCA 2 activation by dietary or pharmacological means instructs Ly-6C Lo monocytes and/or macrophages to deliver a neuroprotective signal to the brain. Glucose and the ketone body β-hydroxybutyrate (BHB) are the brain’s energy substrates. An energy deficit plays a causal role in ischemic stroke and has also been involved in other neurodegenerative diseases, such as Parkinson’s disease (PD), Alzheimer’s disease (AD) and amyotrophic lateral sclerosis (ALS) [1] , [2] . Therefore, ample supply of glucose and BHB would be expected to ameliorate these diseases. However, the role of glucose and BHB in neurological disorders goes beyond their function as energy substrates. Hyperglycemia aggravates rather than improves ischemic stroke and AD, but the basic mechanisms underlying this paradox are still unclear [3] . BHB does improve various neurological diseases, though not necessarily by supplying extra energy. Over 90 years of clinical experience have shown that ketogenic diet has anticonvulsive efficacy. In clinical practice, ketogenic diet is now established in the treatment of pharmacoresistant childhood epilepsy. In addition, ketogenic diet and BHB exert a protective function in animal models of stroke, PD, AD and ALS [4] , [5] , [6] , [7] , [8] . So far small clinical trials suggest that it is also effective in neurodegenerative diseases [9] . Currently, larger trials are underway to test ketogenic diet in neurodegenerative diseases ( clinicaltrials.gov accession codes NCT01035710, NCT01016522 and NCT01364545). Several mechanisms have been described that explain the antiepileptic efficacy of a ketogenic diet, but the mechanisms underlying its neuroprotective activity have not yet been elucidated [4] , [8] , [10] . It has long been known that BHB produced by the liver from free fatty acids under fasting conditions reduces in a negative feedback loop the release of fatty acids from adipose tissue [11] . This important homeostatic function is believed to be mediated by the hydroxy-carboxylic acid receptor 2 (HCA 2 , GPR109A), a G i protein-coupled receptor that is activated by BHB on adipocytes [12] . Interestingly, HCA 2 is also stimulated by nicotinic acid and related drugs that are in clinical use to lower plasma lipids and protect against atherosclerotic disorders [13] , [14] . HCA 2 is not confined to adipocytes but is also present on neutrophils and tissue macrophages [14] . In addition, expression in the brain has been reported [15] . Therefore, we investigated the function of HCA 2 receptors in the context of neuroprotection induced by ketogenic diet. Our data show that the activation of HCA 2 by ketogenic diet, BHB, or nicotinic acid induces a neuroprotective phenotype in bone marrow-derived macrophages that infiltrate the brain and that this results in an improved outcome in a mouse model of stroke. HCA 2 mediates the neuroprotective effect of ketogenic diet To explore HCA 2 function in ketogenic diet-induced neuroprotection, we employed Hca2 −/− mice. 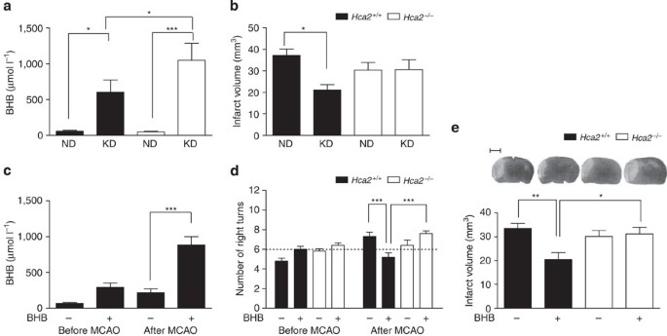Figure 1:HCA2mediates the neuroprotective effect of ketogenic diet and β-hydroxybutyrate. (a) BHB plasma concentrations increased when mice were fed a ketogenic diet (KD). Controls received normal chow (ND). ANOVA, F(3/36)=10.85,P<0.0001. *P<0.05, ***P<0.0001 (Newman–Keulspost hoctest). Values are means±s.e.m. (n=10). (b) Ketogenic diet reduced the infarct volume inHca2+/+but not inHca2−/−animals. The infarct volume was determined 48 h after MCAO. ANOVA, F(3/35)=3.692,P<0.05. *P<0.05 (Newman–Keulspost hoctest). Values are means±s.e.m. (n=9–10). (c) BHB plasma concentrations increased when mice were treated with BHB (8 mg h−1) to similar levels as on ketogenic diet. Measurements were performed immediately before MCAO or 48 h after MCAO. ANOVA, F(3/8)=24.28,P=0.0002. ***P<0.0001 (Newman–Keulspost hoctest). Values are means±s.e.m. (n=3). (d) In the corner test, vehicle-treatedHca2+/+mice showed a preference to turn to the right side 48 h after MCAO. BHB treatment reduced this preference for right turns. BHB-treatedHca2−/−mice had a higher tendency for right turns thanHca2+/+mice after MCAO. The dashed line indicates the expected behaviour without a side preference in 12 trials of the corner test. Two-way repeated-measures ANOVA, F(3/36)=5.154,P=0.0046. ***P<0.001 (Bonferronipost hoctest). Values are means±s.e.m. (n=10). (e) BHB treatment reduced the infarct volume inHca2+/+but not inHca2−/−mice. The infarct volume was determined 48 h after MCAO. Typical silver-stained coronal brain sections showing infarcts in light grey are depicted on top of the panel. For vehicle treatment, pumps filled with saline were implanted. ANOVA, F(3/36)=4.909,P=0.0058. *P<0.05, **P<0.01 (Newman–Keulspost hoctest). Values are means±s.e.m. (n=10). Scale bar, 2.5 mm. When we fed wild-type ( Hca2 +/+ ) or Hca2 −/− mice with a ketogenic diet, body weight did not change ( Supplementary Table 1 ) but plasma concentrations of BHB increased markedly ( Fig. 1a ). In keeping with the concept that, HCA 2 provides a negative feedback on ketone body production by inhibiting fatty acid release [11] , [12] , the BHB levels were even higher in Hca2 −/− than in wild-type mice ( Fig. 1a ). Plasma levels of free fatty acids and acetoacetate increased similarly ( Supplementary Table 1 ). We induced ischemic strokes by occluding the distal middle cerebral artery (MCAO). This procedure induces mainly cortical infarcts. Forty-eight hours after MCAO, infarcts were significantly smaller in wild-type mice on a ketogenic diet than in animals on a normal diet ( Fig. 1b ). Interestingly, the protective effect of the diet was lost in Hca 2 −/− mice, although they had higher plasma levels of ketone bodies ( Fig. 1a,b ; Supplementary Table 1 ). However, there was no significant difference in the infarct size between the genotypes when mice were fed a normal diet. Figure 1: HCA 2 mediates the neuroprotective effect of ketogenic diet and β-hydroxybutyrate. ( a ) BHB plasma concentrations increased when mice were fed a ketogenic diet (KD). Controls received normal chow (ND). ANOVA, F (3/36) =10.85, P <0.0001. * P <0.05, *** P <0.0001 (Newman–Keuls post hoc test). Values are means±s.e.m. ( n =10). ( b ) Ketogenic diet reduced the infarct volume in Hca2 +/+ but not in Hca2 −/− animals. The infarct volume was determined 48 h after MCAO. ANOVA, F(3/35)=3.692, P <0.05. * P <0.05 (Newman–Keuls post hoc test). Values are means±s.e.m. ( n =9–10). ( c ) BHB plasma concentrations increased when mice were treated with BHB (8 mg h −1 ) to similar levels as on ketogenic diet. Measurements were performed immediately before MCAO or 48 h after MCAO. ANOVA, F (3/8) =24.28, P =0.0002. *** P <0.0001 (Newman–Keuls post hoc test). Values are means±s.e.m. ( n =3). ( d ) In the corner test, vehicle-treated Hca2 +/+ mice showed a preference to turn to the right side 48 h after MCAO. BHB treatment reduced this preference for right turns. BHB-treated Hca2 −/− mice had a higher tendency for right turns than Hca2 +/+ mice after MCAO. The dashed line indicates the expected behaviour without a side preference in 12 trials of the corner test. Two-way repeated-measures ANOVA, F (3/36) =5.154, P =0.0046. *** P <0.001 (Bonferroni post hoc test). Values are means±s.e.m. ( n =10). ( e ) BHB treatment reduced the infarct volume in Hca2 +/+ but not in Hca2 −/− mice. The infarct volume was determined 48 h after MCAO. Typical silver-stained coronal brain sections showing infarcts in light grey are depicted on top of the panel. For vehicle treatment, pumps filled with saline were implanted. ANOVA, F (3/36) =4.909, P =0.0058. * P <0.05, ** P <0.01 (Newman–Keuls post hoc test). Values are means±s.e.m. ( n =10). Scale bar, 2.5 mm. Full size image BHB is the endogenous ligand of HCA 2 receptors [12] . To test whether BHB is involved in reducing the infarct size via HCA 2 receptors, we administered BHB by implanting subcutaneous pumps because of its short half-life. This treatment elevated plasma levels of BHB 48 h after MCAO ( Fig. 1c ). In parallel, BHB treatment improved the stroke-induced neurological deficit as shown by the corner test. In 12 trials, mice tended to turn more often to the contralateral (that is, right) than to the ipsilateral side after MCAO. BHB treatment normalized this preference for the right side in wild-type but not in Hca2 −/− mice ( Fig. 1d ). Furthermore, BHB decreased the infarct volume in wild-type but not in Hca2 −/− animals, demonstrating a neuroprotective effect of BHB through HCA 2 receptors ( Fig. 1e ; Supplementary Fig. 1 ). Nicotinic acid mimics the effect of ketogenic diet HCA 2 is activated by nicotinic acid, a drug that is used clinically to lower serum lipid concentrations [13] . In doses equal or lower than those used before in mice to exert clinically relevant effects [16] , [17] , nicotinic acid reduced the infarct size and the ischemic disruption of the blood–brain barrier ( Fig. 2a,b ). 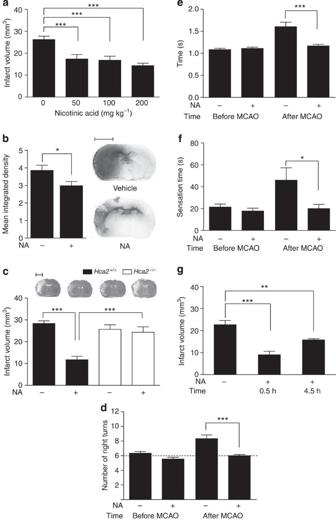Figure 2:The HCA2agonist nicotinic acid ameliorates the consequences of ischemic stroke. (a) Nicotinic acid at doses similar to those used in the clinic reduced the infarct volume. The infarct volume was determined 48 h after MCAO. ANOVA, F(3/103)=12.68,P<0.0001. ***P<0.0001 (Newman–Keulspost hoctest). (b) In parallel, the extravasation of IgG into the ischemic area was reduced by nicotinic acid treatment (NA, 100 mg kg−1). The IgG content was measured 48 h after MCAO by immunohistochemistry. *P<0.05 (t-test). Values are means±s.e.m. (n=11). Scale bar, 2.5 mm. (c) The protective effect of nicotinic acid (100 mg kg−1) was lost inHca2−/−mice. The infarct volume was determined 48 h after MCAO. Typical silver-stained coronal brain sections showing infarcts in light grey are depicted on top of the panel. ANOVA, F(3/48)=15.81,P<0.0001. ***P<0.0001 (Newman–Keulspost hoctest). Values are means±s.e.m. (n=12–14). Scale bar, 2.5 mm. (d) In the corner test, nicotinic acid treatment (100 mg kg−1) improved the preference that was observed in vehicle-treated animals to turn to the right side 48 h after MCAO. The dashed line indicates the expected behaviour without a side preference in 12 trials of the corner test. Two-way repeated-measures ANOVA, F(1/16)=20.36,P=0.0004. ***P<0.001 (Bonferronipost hoctest). Values are means±s.e.m. (n=9). (e) Nicotinic acid treatment (100 mg kg−1) improved the latency to move that was increased 48 h after MCAO. Two-way repeated-measures ANOVA, F(1/15)=13.30,P=0.0024. ***P<0.001 (Bonferronipost hoctest). Values are means±s.e.m. (n=8–9). (f) After nicotinic acid treatment (100 mg kg−1) mice started removing sticky tape fixed to the right front paw earlier. Nicotinic acid treatment only started 30 min after MCAO with the dosing intervals specified in the Methods section. The behavioural test was performed 48 h after MCAO. Two-way repeated-measures ANOVA, F(1/18)=11.28,P<0.05. *P<0.05 (Bonferronipost hoctest). Values are means±s.e.m. (n=10). (g) Nicotinic acid (100 mg kg−1) reduced the infarct volume when administered 30 min or 4.5 h after MCAO. The infarct volume was determined 48 h after MCAO. ANOVA, F(2/21)=21.05,P<0.0001. **P<0.001, ***P<0.0001 (Newman–Keulspost hoctest). Values are means±s.e.m. (n=8). Physiological parameters that are known to influence the infarct volume, such as mean arterial blood pressure, blood gases and body temperature were not affected by nicotinic acid treatment ( Supplementary Table 2 ). Laser Doppler flow measurements showed that nicotinic acid did not significantly change cerebral blood flow, although the measurement at a single site may have missed localized effects. Only blood glucose concentrations increased significantly in response to nicotinic acid, which is in line with clinical experience ( Supplementary Table 2 ). However, hyperglycaemia is more likely to diminish the neuroprotective effect of nicotinic acid because elevated glucose concentrations increase the infarct volume in this and in other stroke models [3] . When we repeated the experiment in wild-type and Hca2 −/− mice, nicotinic acid was only effective in wild-type but not in Hca2 −/− mice, demonstrating that by activating HCA 2 a neuroprotective effect is produced ( Fig. 2c ). Importantly, nicotinic acid also improved the stroke-induced neurological deficit that was evaluated by three established tests of sensorimotor function [18] . In the corner test, nicotinic acid treatment normalized the preference for the right side ( Fig. 2d ). After MCAO, the latency to move one body length was prolonged. Nicotinic acid treatment significantly improved this parameter ( Fig. 2e ). Finally, in the sticky-tape-removal test, mice needed more time to sense the tape on the contralateral forepaw after MCAO. Nicotinic acid treatment also reduced the time needed to complete this test ( Fig. 2f ). Figure 2: The HCA 2 agonist nicotinic acid ameliorates the consequences of ischemic stroke. ( a ) Nicotinic acid at doses similar to those used in the clinic reduced the infarct volume. The infarct volume was determined 48 h after MCAO. ANOVA, F (3/103) =12.68, P <0.0001. *** P <0.0001 (Newman–Keuls post hoc test). ( b ) In parallel, the extravasation of IgG into the ischemic area was reduced by nicotinic acid treatment (NA, 100 mg kg −1 ). The IgG content was measured 48 h after MCAO by immunohistochemistry. * P <0.05 ( t -test). Values are means±s.e.m. ( n =11). Scale bar, 2.5 mm. ( c ) The protective effect of nicotinic acid (100 mg kg −1 ) was lost in Hca2 −/− mice. The infarct volume was determined 48 h after MCAO. Typical silver-stained coronal brain sections showing infarcts in light grey are depicted on top of the panel. ANOVA, F (3/48) =15.81, P <0.0001. *** P <0.0001 (Newman–Keuls post hoc test). Values are means±s.e.m. ( n =12–14). Scale bar, 2.5 mm. ( d ) In the corner test, nicotinic acid treatment (100 mg kg −1 ) improved the preference that was observed in vehicle-treated animals to turn to the right side 48 h after MCAO. The dashed line indicates the expected behaviour without a side preference in 12 trials of the corner test. Two-way repeated-measures ANOVA, F (1/16) =20.36, P =0.0004. *** P <0.001 (Bonferroni post hoc test). Values are means±s.e.m. ( n =9). ( e ) Nicotinic acid treatment (100 mg kg −1 ) improved the latency to move that was increased 48 h after MCAO. Two-way repeated-measures ANOVA, F (1/15) =13.30, P =0.0024. *** P <0.001 (Bonferroni post hoc test). Values are means±s.e.m. ( n =8–9). ( f ) After nicotinic acid treatment (100 mg kg −1 ) mice started removing sticky tape fixed to the right front paw earlier. Nicotinic acid treatment only started 30 min after MCAO with the dosing intervals specified in the Methods section. The behavioural test was performed 48 h after MCAO. Two-way repeated-measures ANOVA, F (1/18) =11.28, P <0.05. * P <0.05 (Bonferroni post hoc test). Values are means±s.e.m. ( n =10). ( g ) Nicotinic acid (100 mg kg −1 ) reduced the infarct volume when administered 30 min or 4.5 h after MCAO. The infarct volume was determined 48 h after MCAO. ANOVA, F (2/21) =21.05, P <0.0001. ** P <0.001, *** P <0.0001 (Newman–Keuls post hoc test). Values are means±s.e.m. ( n =8). Full size image In the experiments described so far, nicotinic acid treatment started immediately before MCAO. However, in clinical practice treatment of stroke is often delayed. Therefore, we administered nicotinic acid after onset of MCAO. Although the delayed dosage reduced the efficacy, nicotinic acid still decreased the infarct size significantly when administered up to 4.5 h after MCAO ( Fig. 2g ). Cellular localization of HCA 2 in the ischemic brain To localize HCA 2 expression in the brain, we used the BAC-transgenic mouse line Hca2 mRFP ( Gpr109a mRFP ), in which the Hca2 locus directs the expression of the monomeric red fluorescent protein (mRFP) [17] . Under normal conditions, mRFP was expressed exclusively by CD11b + microglia, but not by astrocytes and neurons ( Fig. 3a–c ). After MCAO, mRFP + cells accumulated in the periphery of the cortical ischemia ( Fig. 3d ). They expressed CD11b (87.5±14.6% of mRFP + cells) and Iba1 (98.7±18.0% of mRFP + cells), indicating that HCA 2 is present on microglia or monocytes/macrophages that infiltrated the ischemic brain. To differentiate these two cell populations, we generated chimeric mice by transplanting wild-type bone marrow to Hca2 mRFP mice (WT> Hca2 mRFP ) and Hca2 mRFP bone marrow to wild-type mice ( Hca2 mRFP >WT). The analysis of WT> Hca2 mRFP mice revealed that brain-derived mRFP + cells that were CD11b + and correspond to microglia accumulated in the periphery of the infarct ( Fig. 3e ). In addition, we found evidence that bone marrow-derived monocytes/macrophages express HCA 2 in the ischemic brain. In Hca2 mRFP >WT animals, numerous bone marrow-derived mRFP + cells were found in the periphery of the ischemia, whereas scarce mRFP + cells were present in the nonischemic hemisphere ( Fig. 3f ). Bone marrow-derived mRFP + cells expressing CD11b were already detected 24 h after MCAO in the ischemic brain of Hca2 mRFP >WT mice, but their number was higher 48 h after MCAO ( Figs 3g and 4a–e ). A further analysis by flow cytometry demonstrated that most mRFP + cells in the ischemic hemisphere were CD11b + , CD45 + and Ly-6G − suggesting a monocytic/macrophagic identity ( Fig. 4a–g ). As reported previously [19] , Ly-6C Hi and Ly-6C Lo monocytes/macrophages were present in the ischemic area representing an inflammatory and a resident subset of monocytes/macrophages, respectively [20] ( Fig. 4f,g ). Interestingly, mRFP + monocytes/macrophages in the ischemic brain were mainly of a Ly-6C Lo subtype ( Fig. 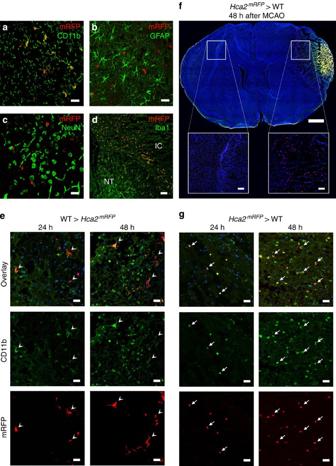Figure 3:Microglia and monocytes or macrophages infiltrating the ischemic brain express HCA2. (a–c) Evidence for the expression of HCA2in CD11b+microglia under normal conditions. InHca2mRFPmice, mRFP (red) reflects HCA2expression. CD11b, the astrocyte marker GFAP, and the neuronal marker NeuN were detected by immunohistochemistry. Scale bar, 20 μm. (d) InHca2mRFPmice, mRFP+cells markedly increased in the periphery of the ischemic area 48 h after MCAO. Most mRFP+cells expressed Iba1, a marker of microglia and infiltrating monocytes/macrophages. IC, ischemic core. NT, normal tissue. Scale bar, 100 μm. (e) When wild-type bone marrow was transplanted toHca2mRFP(WT>Hca2mRFP), mRFP+cells (red) that were stained with anti-CD11b (green) were found in the periphery of the ischemic area 24 h and 48 h after MCAO. The double-positive cells (white arrowheads) had several processes in accordance with their microglial identity. Images are representative for results obtained in three chimeric mice. Scale bar, 25 μm. (f) WhenHca2mRFPbone marrow was transplanted to wild-type mice (Hca2mRFP>WT), mRFP+cells (red) accumulated in the periphery of the ischemic area 48 h after MCAO. The yellow fluorescent signal in the core of the infarct was due to autofluorescence. Scale bar in the overview, 500 μm. Scale bar in the insets, 100 μm. (g) InHca2mRFP>WT mice, mRFP+cells (red) were stained with anti-CD11b (green, white arrows) and increased in number between 24 h and 48 h after MCAO. Images are representative for results obtained in three chimeric mice per time point. Scale bar, 25 μm. 4f,g ; Supplementary Table 3 ). In contrast, in blood mRFP + CD45 + CD11b + Ly-6G − monocytes spread equally between Ly-6C Lo and Ly-6C Hi subsets before MCAO ( Fig. 5 ). After MCAO, the number of Ly-6C Hi monocytes dropped but Ly-6C Lo monocytes remained stable. This suggests that HCA 2 -expressing Ly-6C Lo monocytes preferentially infiltrate the ischemic brain or, more likely in view of previous data [19] , that Ly-6C Hi cells differentiate into this cell type. Figure 3: Microglia and monocytes or macrophages infiltrating the ischemic brain express HCA 2 . ( a – c ) Evidence for the expression of HCA 2 in CD11b + microglia under normal conditions. In Hca2 mRFP mice, mRFP (red) reflects HCA 2 expression. CD11b, the astrocyte marker GFAP, and the neuronal marker NeuN were detected by immunohistochemistry. Scale bar, 20 μm. ( d ) In Hca2 mRFP mice, mRFP + cells markedly increased in the periphery of the ischemic area 48 h after MCAO. Most mRFP + cells expressed Iba1, a marker of microglia and infiltrating monocytes/macrophages. IC, ischemic core. NT, normal tissue. Scale bar, 100 μm. ( e ) When wild-type bone marrow was transplanted to Hca2 mRFP (WT> Hca2 mRFP ), mRFP + cells (red) that were stained with anti-CD11b (green) were found in the periphery of the ischemic area 24 h and 48 h after MCAO. The double-positive cells (white arrowheads) had several processes in accordance with their microglial identity. Images are representative for results obtained in three chimeric mice. Scale bar, 25 μm. ( f ) When Hca2 mRFP bone marrow was transplanted to wild-type mice ( Hca2 mRFP >WT), mRFP + cells (red) accumulated in the periphery of the ischemic area 48 h after MCAO. The yellow fluorescent signal in the core of the infarct was due to autofluorescence. Scale bar in the overview, 500 μm. Scale bar in the insets, 100 μm. ( g ) In Hca2 mRFP >WT mice, mRFP + cells (red) were stained with anti-CD11b (green, white arrows) and increased in number between 24 h and 48 h after MCAO. Images are representative for results obtained in three chimeric mice per time point. Scale bar, 25 μm. 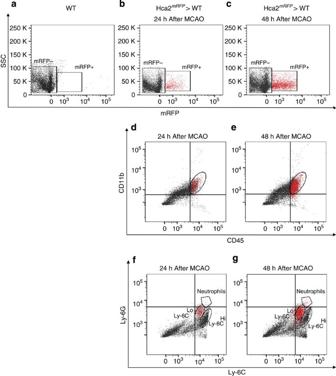Figure 4:Flow cytometric characterization of HCA2-expressing bone marrow-derived cells in the ischemic brain. (a–c) Using flow cytometry after MCAO, we detected mRFP+cells in the brain of chimericHca2mRFP>WT mice but not in wild-type (WT) animals. The number of mRFP+cells increased between 24 h and 48 h after MCAO. For quantification of mRFP+cells seeSupplementary Table 3.Hca2mRFP>WT mice were generated by transplantingHca2mRFPbone marrow to WT animals. (d,e) Gated mRFP+(red dots) and mRFP−(black dots) cells in the ischemic hemisphere were CD11b+CD45+. (f,g) Gated mRFP+cells were mainly Ly-6CLoand Ly-6G−in contrast to mRFP−cells. Only CD45+CD11b+cells are shown. For quantification of cells, seeSupplementary Table 3. Full size image Figure 4: Flow cytometric characterization of HCA 2 -expressing bone marrow-derived cells in the ischemic brain. ( a – c ) Using flow cytometry after MCAO, we detected mRFP + cells in the brain of chimeric Hca2 mRFP >WT mice but not in wild-type (WT) animals. The number of mRFP + cells increased between 24 h and 48 h after MCAO. For quantification of mRFP + cells see Supplementary Table 3 . Hca2 mRFP >WT mice were generated by transplanting Hca2 mRFP bone marrow to WT animals. ( d , e ) Gated mRFP + (red dots) and mRFP − (black dots) cells in the ischemic hemisphere were CD11b + CD45 + . ( f , g ) Gated mRFP + cells were mainly Ly-6C Lo and Ly-6G − in contrast to mRFP − cells. Only CD45 + CD11b + cells are shown. For quantification of cells, see Supplementary Table 3 . 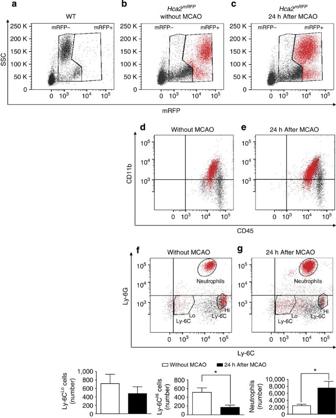Figure 5:Flow cytometric characterization of HCA2-expressing cells in blood. (a–c) We detected mRFP+cells only in the blood ofHca2mRFPmice before and 24 h after MCAO. (d,e) Gated mRFP+(red dots) and mRFP−(black dots) cells were CD11b+CD45+. (f,g) Gated mRFP+cells fell into three populations: Ly-6G+(neutrophils), Ly-6G−Ly-6CLoand Ly-6G−Ly-6CHimonocytes. Only CD45+CD11b+cells are shown. Quantification of mRFP+cells revealed an increase of neutrophils and a decrease of Ly-6CHimonocytes 24 h after MCAO. Values are means±s.e.m. (n=6). *P<0.05 (unpairedt-test). Full size image Figure 5: Flow cytometric characterization of HCA 2 -expressing cells in blood. ( a – c ) We detected mRFP + cells only in the blood of Hca2 mRFP mice before and 24 h after MCAO. ( d , e ) Gated mRFP + (red dots) and mRFP − (black dots) cells were CD11b + CD45 + . ( f , g ) Gated mRFP + cells fell into three populations: Ly-6G + (neutrophils), Ly-6G − Ly-6C Lo and Ly-6G − Ly-6C Hi monocytes. Only CD45 + CD11b + cells are shown. Quantification of mRFP + cells revealed an increase of neutrophils and a decrease of Ly-6C Hi monocytes 24 h after MCAO. Values are means±s.e.m. ( n =6). * P <0.05 (unpaired t -test). Full size image Infiltrating monocytes or macrophages mediate the HCA 2 effect To distinguish whether bone marrow-derived monocytes/macrophages or microglia mediate the protective effect of HCA 2 in stroke, we generated chimeric mice by bone marrow transplantation ( Fig. 6a ). As expected, Hca 2 +/+ mice that received Hca 2 +/+ bone marrow ( Hca2 +/+ > Hca2 +/+ ) were protected by nicotinic acid ( Fig. 6b ). Transplantation of Hca 2 +/+ bone marrow restored the response of Hca2 −/− animals ( Hca2 +/+ > Hca2 −/− ), whereas nicotinic acid lost its activity when Hca2 −/− bone marrow was transplanted to Hca2 +/+ mice ( Hca2 −/− > Hca2 +/+ ), which demonstrates that HCA 2 in bone marrow-derived cells mediates the protective effect of nicotinic acid ( Fig. 6b ). The experiment also showed that HCA 2 expression in cells that do not derive from bone marrow, such as adipocytes, is not required for the neuroprotective effect of nicotinic acid, implying that the inhibition of free fatty acid release from adipocytes and other metabolic effects of nicotinic acid [13] do not contribute to neuroprotection. 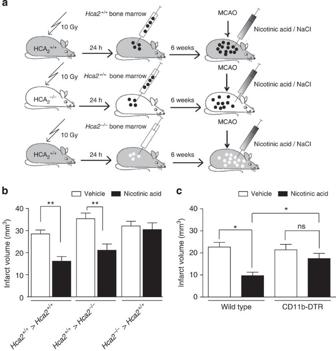Figure 6:Activation of HCA2in bone marrow-derived monocytes/macrophages is neuroprotective. (a) Scheme of the generation of chimeric mice. (b) After transplantingHca2+/+bone marrow to eitherHca2+/+mice (Hca2+/+>Hca2+/+) or toHca2−/−mice (Hca2+/+>Hca2−/−) nicotinic acid (100 mg kg−1) reduced the infarct size. However, whenHca2−/−bone marrow was transplanted toHca2+/+mice (Hca2−/−>Hca2+/+) nicotinic acid was no longer effective. The infarct volume was measured 48 h after MCAO. ANOVA, F(5/50)=8.454,P<0.0001. **P<0.001 (Newman–Keulspost hoctest). Values are means±s.e.m. (n=9–10). (c) The protective effect of nicotinic acid (100 mg kg−1) was lost when CD11b+cells had been ablated. To ablate CD11b+cells, we treated CD11b-DTR mice with diphtheria toxin as described in Methods. Wild-type mice received the same treatment. The infarct volume was determined 48 h after MCAO. ANOVA, F(3/32)=7.038,P<0.001. *P<0.05 (Newman–Keulspost hoctest). Values are means±s.e.m. (n=8–10). Figure 6: Activation of HCA 2 in bone marrow-derived monocytes/macrophages is neuroprotective. ( a ) Scheme of the generation of chimeric mice. ( b ) After transplanting Hca2 +/+ bone marrow to either Hca2 +/+ mice ( Hca2 +/+ > Hca2 +/+ ) or to Hca2 −/− mice ( Hca2 +/+ > Hca2 −/− ) nicotinic acid (100 mg kg −1 ) reduced the infarct size. However, when Hca2 −/− bone marrow was transplanted to Hca2 +/+ mice ( Hca2 −/− > Hca2 +/+ ) nicotinic acid was no longer effective. The infarct volume was measured 48 h after MCAO. ANOVA, F (5/50) =8.454, P <0.0001. ** P <0.001 (Newman–Keuls post hoc test). Values are means±s.e.m. ( n =9–10). ( c ) The protective effect of nicotinic acid (100 mg kg −1 ) was lost when CD11b + cells had been ablated. To ablate CD11b + cells, we treated CD11b-DTR mice with diphtheria toxin as described in Methods. Wild-type mice received the same treatment. The infarct volume was determined 48 h after MCAO. ANOVA, F (3/32) =7.038, P <0.001. * P <0.05 (Newman–Keuls post hoc test). Values are means±s.e.m. ( n =8–10). Full size image To further define the bone marrow-derived cell type that is responsible for the effect of nicotinic acid, we used CD11b-DTR mice that express the human diphtheria toxin receptor under control of the CD11b promoter [21] . In these mice treatment with diphtheria toxin (DT) ablated blood monocytes/macrophages but not neutrophils [19] , [21] . After DT treatment, the number of CD11b + cells in peripheral blood of CD11b-DTR mice was reduced by 92% in comparison with wild-type animals. As reported previously, ablation of CD11b + cells by itself did not alter the infarct size ( Fig. 6c ) [19] . However, when monocytes/macrophages had been ablated, nicotinic acid no longer reduced the infarct volume ( Fig. 6c ), demonstrating that the neuroprotective effect of nicotinic acid depends on monocytes/macrophages. PGD 2 is responsible for the neuroprotective effect of HCA 2 The activation of HCA 2 by nicotinic acid or other agonists is known to stimulate the synthesis of PGD 2 (ref. 14 ). In the skin, PGD 2 is responsible for the flushing response induced by nicotinic acid. In the brain, however, PGD 2 exerts neuroprotective effects [22] . Therefore, we investigated whether PGD 2 production mediates the neuroprotective effect of HCA 2 activation. Haematopoietic PGD 2 synthase (HPGDS) and COX1 are responsible for synthesizing PGD 2 and its derivatives in macrophages [23] , [24] . In accordance with the finding that, HCA 2 activation stimulates PGD 2 release from macrophages [25] , plasma concentrations of PGD 2 and the renal excretion of tetranor PGDM, a major PGD 2 metabolite that reflects the synthesis of PGD 2 (ref. 26 ), increased on nicotinic acid treatment ( Fig. 7a,d ). Nicotinic acid is able to penetrate the blood–brain barrier [27] . Twenty-four hours after MCAO, when monocytes/macrophages have infiltrated the ischemic area, we also found elevated PGD 2 concentrations in the brain on the activation of HCA 2 by nicotinic acid ( Fig. 7b ). To test the role of PGD 2 synthesis in HCA 2 -mediated neuroprotection, we used Cox1 −/− mice and an inhibitor of HPGDS. In our stroke model, the infarct volume in vehicle-treated Cox1 −/− mice was similar as in Cox1 +/+ animals in line with some but not all previous studies ( Fig. 7c ) [28] , [29] , [30] . Interestingly, nicotinic acid had no effect on the infarct volume in Cox1 −/− mice, whereas Cox1 +/+ littermates were protected ( Fig. 7c ). When we inhibited HPGDS in mice with the small molecule compound HQL79 (ref. 31 ), renal excretion of the PGD 2 metabolite tetranor PGDM was reduced confirming the efficacy of HQL79 as a HPGDS inhibitor ( Fig. 7d ). In parallel, the protective effect of nicotinic acid was partially reversed by HQL79 ( Fig. 7e ), suggesting that COX1 and HPGDS mediate the effect of nicotinic acid. 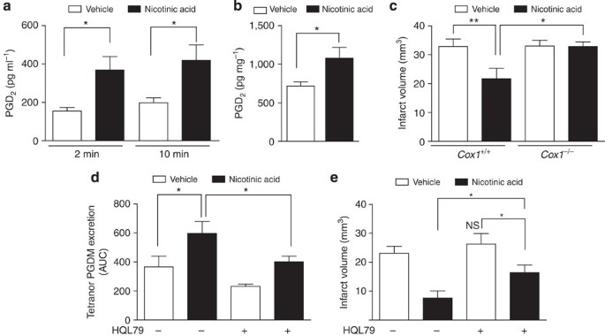Figure 7:HCA2activation by nicotinic acid depends on COX1 and the haematopoietic PGD2synthase (HPGDS). (a) PGD2plasma concentrations increased after nicotinic acid treatment. The time between nicotinic acid (100 mg kg−1) treatment and blood sampling is indicated. Two-way repeated-measures ANOVA, F(1/15)=16.45,P=0.001. *P<0.05 (Bonferronipost hoctest). Values are means±s.e.m. (n=8–9). (b) In the brain, PGD2concentrations increased 24 h after MCAO when nicotinic acid was injected 5 min before extraction. *P<0.05 (ttest,n=6–7). (c) The protective effect of nicotinic acid (100 mg kg−1) was lost inCox1−/−mice. The infarct volume was determined 48 h after MCAO. ANOVA, F(3/30)=4.617,P<0.01. *P<0.05, **P<0.001 (Newman–Keulspost hoctest). Values are means±s.e.m. (n=7–8). (d) Urinary excretion of the PGD2metabolite tetranor PGDM was stimulated by nicotinic acid treatment (100 mg kg−1). HQL79 (30 mg kg−1) reduced the excretion of tetranor PGDM. Values are means±s.e.m. (n=10–11) of the area under the concentration-time curve (AUC) for tetranor PGDM in urine. Tetranor PGDM was measured at hourly intervals for 4 h after nicotinic acid administration. ANOVA, F(3/38)=7.041,P<0.001. *P<0.05 (Newman–Keulspost hoctest). (e) Inhibition of HPGDS by HQL79 (30 mg kg−1) partially reversed the neuroprotective effect of nicotinic acid (100 mg kg−1). Infarct volumes were determined 48 h after MCAO. ANOVA, F(3/36)=8.471.P=0.0002. *P<0.05 (Newman–Keulspost hoctest). NS, nonsignificant in comparison with the group without HQL79 and nicotinic acid. Values are means±s.e.m. (n=10). Figure 7: HCA 2 activation by nicotinic acid depends on COX1 and the haematopoietic PGD 2 synthase (HPGDS). ( a ) PGD 2 plasma concentrations increased after nicotinic acid treatment. The time between nicotinic acid (100 mg kg −1 ) treatment and blood sampling is indicated. Two-way repeated-measures ANOVA, F (1/15) =16.45, P =0.001. * P <0.05 (Bonferroni post hoc test). Values are means±s.e.m. ( n =8–9). ( b ) In the brain, PGD 2 concentrations increased 24 h after MCAO when nicotinic acid was injected 5 min before extraction. * P <0.05 ( t test, n =6–7). ( c ) The protective effect of nicotinic acid (100 mg kg −1 ) was lost in Cox1 −/− mice. The infarct volume was determined 48 h after MCAO. ANOVA, F (3/30) =4.617, P <0.01. * P <0.05, ** P <0.001 (Newman–Keuls post hoc test). Values are means±s.e.m. ( n =7–8). ( d ) Urinary excretion of the PGD 2 metabolite tetranor PGDM was stimulated by nicotinic acid treatment (100 mg kg −1 ). HQL79 (30 mg kg −1 ) reduced the excretion of tetranor PGDM. Values are means±s.e.m. ( n =10–11) of the area under the concentration-time curve (AUC) for tetranor PGDM in urine. Tetranor PGDM was measured at hourly intervals for 4 h after nicotinic acid administration. ANOVA, F (3/38) =7.041, P <0.001. * P <0.05 (Newman–Keuls post hoc test). ( e ) Inhibition of HPGDS by HQL79 (30 mg kg −1 ) partially reversed the neuroprotective effect of nicotinic acid (100 mg kg −1 ). Infarct volumes were determined 48 h after MCAO. ANOVA, F (3/36) =8.471. P =0.0002. * P <0.05 (Newman–Keuls post hoc test). NS, nonsignificant in comparison with the group without HQL79 and nicotinic acid. Values are means±s.e.m. ( n =10). Full size image Ketogenic diet and BHB are known to protect against seizures and neurodegeneration. Here we provide evidence that the neuroprotective action of ketogenic diet and of the endogenous ketone body BHB is mediated by HCA 2 . BHB activates HCA 2 with an EC 50 of ~\n750 μM (ref. 32 ), similar to the BHB plasma concentrations of 600–1,000 μM ( Fig. 1a,c ) that we found to be associated with neuroprotection. In contrast, higher BHB concentrations are required in vitro to protect neurons lacking HCA 2 (refs 33 , 34 , 35 ). While in our experiments neuroprotection coincided with elevated BHB levels, anti-seizure effects seem to lag behind ketosis [36] , suggesting that the neuroprotective and the anti-seizure effects are mediated by different mechanisms. Previous studies showed that HCA 2 is activated on adipocytes by BHB and the anti-dyslipidemic drug nicotinic acid [12] , [14] . However, the potential of HCA 2 to improve CNS disorders was unknown. We found that under normal conditions, microglia express HCA 2 . Nevertheless, our experiments employing bone marrow transplantation argue against a major role of microglia in HCA 2 -induced neuroprotection because this cell population is not exchanged by bone marrow transplantation [37] . Among bone marrow-derived cells, neutrophils and monocytes/macrophages express HCA 2 (ref. 14 ). The activation of HCA 2 inhibits adhesion and migration of neutrophils and induces the death of these cells in vitro [38] , [39] . Whether modulation of neutrophils contributes to the neuroprotective effects of HCA 2 in cerebral ischemia is still unclear. However, the neuroprotective effect of HCA 2 depended on monocytes/macrophages ( Fig. 6c ) that infiltrate the brain in ischemic stroke [19] . Interestingly, HCA 2 was found on a subset of immigrant monocytes/macrophages that was characterized by low expression of Ly-6C, demonstrating that they represent resident monocytes/macrophages [20] . Recently, this noninflammatory type of monocytes/macrophages has been implicated in protection and repair in stroke and other diseases [15] , [18] , [40] . Our data suggest that HCA 2 provides a way to specifically activate Ly-6C Lo resident monocytes/macrophages in brain pathology. So far it is unclear whether HCA 2 activates Ly-6C Lo monocytes/macrophages before brain infiltration in blood or in the ischemic brain. However, the observations that nicotinic acid is able to penetrate into the brain [27] and that nicotinic acid treatment leads to elevated PGD 2 levels in the brain argue for an effect within the CNS. The protective effect of HCA 2 activation depended on COX1 and HPGDS, the key enzymes that synthesize PGD 2 in response to nicotinic acid treatment [17] , [41] . While we cannot exclude the possible involvement of COX2 or other arachidonic acid products, our data suggest a new concept by which PGD 2 release from monocytes/macrophages mediates the neuroprotective effect of HCA 2 . Previous work has shown that PGD 2 helps to resolve inflammation [42] . In addition, it has neuroprotective effects [22] , [43] . PGD 2 has a short half-life in tissue and is spontaneously converted into the cyclopentenone 15-deoxy-Δ 12,14 -prostaglandin J 2 (15d-PGJ 2 ), which inhibits the IκB kinase (IKK), the main activator of the transcription factor NF-κB and a key player in ischemic brain damage [44] , [45] . In accordance with this, HCA 2 activation has been shown to inhibit NF-κB activation in bone marrow-derived macrophages [46] . 15d-PGJ 2 is also an endogenous agonist of PPARγ, a transcription factor with neuroprotective properties [47] , [48] . Via this mechanism, nicotinic acid is able to stimulate PPARγ in human monocytes in vitro [24] . Furthermore, it has been reported that 15d-PGJ 2 can stimulate angiogenesis [49] . Similar mechanisms may underlie the anti-atherogenic effect of HCA 2 activation [50] . In vascular macrophages, HCA 2 activation upregulated genes with an anti-inflammatory and anti-atherogenic function [50] . Collectively, these data suggest that HCA 2 provides the pharmacological basis to modulate monocyte/macrophage function and to redirect these cells into a salutary pathway. Our study demonstrates that HCA 2 activation induces a neuroprotective repertoire of resident monocytes/macrophages that can reduce ischemic brain damage. Infiltration of monocytes/macrophages into the diseased brain has also been noted in chronic neurodegenerative disorders, such as AD, PD and ALS, and MS [51] , [52] , [53] , which suggests that the findings we obtained in a model of ischemic stroke may have implications that extend beyond this specific disease. In line with this notion, ketogenic diet and the subsequent production of the endogenous HCA 2 agonist BHB are effective in the treatment of several chronic neurodegenerative disorders [9] . However, compliance is often low because the diet is unpalatable. The discovery of the central role of HCA 2 may guide drug development and may ultimately lead to a ‘ketogenic diet in a pill’ [10] . Importantly, the HCA 2 receptor is a good target for drug development. The prototypical agonist nicotinic acid has been known to ameliorate ischemic brain damage [54] , [55] . More than 50 years ago, before the era of evidence-based medicine, it was used in human stroke patients because of its vasodilatory effects that are apparent from the flushing response in the face [56] , [57] , [58] . However, later studies found little or no vasodilatory effect in cerebral vessels [59] , [60] . Thus, its mode of action had been largely unclear. Our data now demonstrate that the neuroprotective activity of nicotinic acid depends on HCA 2 , very much as that of BHB and ketogenic diet. HCA 2 may also mediate the protective effect of dimethyl fumarate and its metabolite monomethyl fumarate in multiple sclersosis [38] , [61] . Novel HCA 2 agonists showed evidence of a superior potency or of fewer side effects than nicotinic acid during clinical trials testing anti-dyslipidemic effects [16] , [62] , [63] . Thus, synthetic HCA 2 agonists provide the pharmacological basis for modulating monocyte/macrophage function and redirecting these important cells into a neuroprotective pathway. Mice Hca2 −/− , Hca2 mRFP (Gpr109a mRFP ), CD11b-DTR, and Cox1 −/− mice have been reported previously [13] , [17] , [21] , [64] . The Hca2 −/− mice were backcrossed for more than eight generations on a C57BL/6 background; therefore, we used C57BL/6 mice as wild-type controls. To habituate mice to ketogenic diet (sniff EF R/M ketogenic diet with 80% long-chain fatty acids in dry mass and 8% protein), we mixed it with normal chow (ssniff M-Z, containing 48% carbohydrates, 15% fat and 37% protein) and increased the fraction of ketogenic diet in a stepwise manner (50% for 3 days, 70% for 5 days, 90% for 6 days and 100% for 4 days). All experiments were performed according to the German animal protection law and approved by the local animal welfare authorities (Regierungspräsidium Karlsruhe; Ministerium für Energiewende, Landwirtschaft, Umwelt und ländliche Räume, Kiel, Germany). Stroke model In the model, 8- to 15-week-old male mice were subjected to left middle cerebral artery occlusion (MCAO) as described previously [65] . In brief, the mice were anaesthetized with 15 μl 2.5% tribromoethanol per gram body weight. Panthenol eye ointment was used to prevent eye dryness. A skin incision was made between the ear and the orbit on the left side. The temporal muscle was removed and a burr hole was drilled to expose the stem of the middle cerebral artery (MCA). The MCA was then occluded by microbipolar electrocoagulation (Modell ICC 50, Erbe, Tübingen, Germany). The surgery was done under a microscope (Hund, Wetzlar, Germany), and rectal temperature was maintained at 37 °C during surgery by a heating pad. The skin incision was then closed by suture, and the mice were placed under a heating lamp until they fully recovered. After 24 or 48 h of MCAO, mice were deeply reanaesthetized with tribromoethanol and perfused intracardially with 15 to 20 ml of Ringer’s solution. Brains were carefully removed and coronally cryosectioned (20-μm thick) every 400 μm. Coronal sections were then stained with a silver technique [18] , and the infarct volume was determined using ImageJ and corrected for brain edema as described previously [18] , [45] . Mice were only excluded from analysis if they died before perfusion. The mortality of mice that underwent surgery was 7.6%. To analyse physiological parameters, the femoral artery was cannulated in a separate cohort of animals. Blood samples (100 μl) were withdrawn 10 min before and 10 min after the MCAO. Investigators were blinded to the treatment or genotype of mice or to both in all experiments. Mice were randomized to the treatment groups. If not indicated otherwise, nicotinic acid or vehicle was administered 10 min before MCAO and 4 h, 8 h, 24 h, 28 h and 32 h after MCAO. Because of its short half-life, we administered BHB through subcutaneous Alzet pumps (2001D, releasing 8 μl h −1 BHB, 1 g ml −1 , dissolved in normal saline) that were implanted subcutaneously 10 h before MCAO under isoflurane anaesthesia; controls received pumps filled with normal saline. HQL79 was suspended in Methocel (0.2 ml, 0.5%) and administered by gavage 1 h before each nicotinic acid dose. Controls received the vehicle by gavage. Bone marrow transplantation and ablation of CD11b-positive cells Bone marrow transplantation was performed as described previously [66] with the following modifications. Mice were killed by cervical dislocation, and bone marrow was aseptically collected from femurs and tibias. Unfractionated bone marrow cells were resuspended in 0.25 ml sterile PBS and injected retro-orbitally into 10- to 13-week-old C57BL/6, Hca2 −/− , or Hca2 mRFP mice that had been lethally irradiated (dose of 10 Gy in 2 divided sessions, 5 Gy each time with a 4-h interval, 10 MV- bremsstrahlung, dose rate of 3 Gy min −1 ) 1 day before. Six weeks after reconstitution, mice were subjected to MCAO. To ablate CD11b + cells, we injected CD11b-DTR mice with diphtheria toxin (ip, 25 ng g −1 body weight) 48 h and 24 h before MCAO. Wild-type controls were also treated with diphtheria toxin. Behavioural analysis To evaluate sensorimotor function, we used three established tests. The corner and latency-to-move test have been described previously [18] . In brief, mice were allowed to enter a 30 × 20-cm corner with an angle of 30° before and 48 h after MCAO, and the number of right and left turns on rearing out of 12 trials were counted. For the latency-to-move test, mice were placed at the centre of a plain board. The time to cross one body length (7 cm) was measured before and 48 h after MCAO. In the sticky-tape-removal test, a small circular adhesive tape (HERMA No 2212, 8 mm) was placed onto both forepaws one after another before and 48 h after MCAO, and the time when mice first tried to remove the adhesive tape as well as the total time needed to remove it were determined. In this study, mice were trained before MCAO three times in 3 days, and the last training session was considered as the baseline value. Flow cytometry Flow cytometry was performed as described previously [67] with the following modifications. Mice were deeply anaesthetized with tribromoethanol 24 h or 48 h after MCAO and perfused intracardially with Ringer’s solution. Brains were dissected and olfactory bulbs, right hemispheres and cerebella were removed. Left hemispheres were digested in DMEM (Invitrogen) containing collagenase A (1 mg ml −1 , Roche) and DNAse (0.1 mg ml −1 , Roche) for 30 min at 37°. Then, cells were filtered through a 40-μm nylon cell strainer (BD Biosciences), and the red blood cells were lysed on ice with standard erythrocyte lysis buffer. Myelin and debris were separated from the cell using Percoll gradient (GE Healthcare; 78 and 30%). The cells were collected carefully from the interface of the gradient and washed with 10 ml PBS containing 0.5% BSA. After treatment with purified rat anti-mouse CD16/32 (Fc Block, BD Pharmingen, 1:100) for 10 min on ice, cells were incubated with the antibodies and respective isotype controls for 30 min on ice as follows: PerCP-labelled rat anti-mouse CD45 (BD Pharmingen, 1:100), PE-Cy7-labelled rat anti-mouse Ly-6C (BD Pharmingen, 1:100), APC-labelled rat anti-mouse Cd11b (BD Pharmingen, 1:100) and FITC-labelled rat anti-mouse Ly-6G (BD Pharmingen, 1:100). The cells were then sorted on BD FACS Aria III (BD Bioscience, 100 μm nozzle) with the laser lines 488, 561 and 633 nm. Immunohistochemistry Twenty-four or 48 hours after MCAO , Hca2 mRFP mice were deeply anaesthetized with tribromoethanol and perfused with Ringer’s solution and 4% PFA. Then, 20-μm-thick coronal cryosections were permeabilized with 0.3% Triton X-100 in PBS for 30 min and blocked with 5% BSA. The sections were incubated with rabbit anti-mouse Iba1 (Wako, 1:100), rat anti-mouse CD11b (AbD Serotec, 1:100), mouse anti-NeuN (Chemicon, 1:500) and rabbit anti-GFAP (DAKO, 1.500) overnight at 4 °C. We used the following secondary antibodies to visualize the staining using a confocal microscope (SP5, Leica): Alexa 488-labelled donkey anti-rabbit (Invitrogen, 1:400) and Alexa 488-labelled donkey anti-rat (Invitrogen). The sections were then washed with PBS containing DAPI (Sigma, 1: 5,000) and mounted with Mowiol. Quantification of IgG extravasation Cryosections were fixed in 100% acetone for 5 min at −20 °C and incubated for 5 min with 1.5% H 2 O 2 in methanol. After washing, sections were blocked with PBS containing 5% BSA and 0.3% Triton X-100 and incubated with HRP-labelled goat anti-mouse IgG (Santa Cruz) for 1 h. Then, DAB was applied for 5 min according to the manufacturer’s instructions (DAB-Kit, Vector SK-4100). After drying, the sections were mounted with Mowiol. The staining was quantified with ImageJ as integrated density of the ischemic hemisphere relative to the contralateral hemisphere. Measurement of ketone bodies and PGD 2 synthesis. Total ketone bodies (acetoacetate+BHB), BHB, and free fatty acids in plasma were measured photometrically on an Olympus AU 400 analyzer (Beckman Coulter, Krefeld, Germany) using Autokit Total Ketone Bodies, Autokit 3-HB and NEFA C kit from Wako Chemicals GmbH (Neuss, Germany). The acetoacetate concentration was calculated by subtracting the BHB levels from the total ketone body levels. Plasma and brain concentrations of PGD 2 were measured using an ELISA kit (Cayman Chemicals) according to the manufacturer’s instructions. The major PGD 2 metabolite tetranor PGDM was measured in urine by ELISA (Cayman Chemicals) at the time of nicotinic acid treatment (baseline level) and four times afterwards at hourly intervals. Tetranor PGDM concentrations were normalized for creatinine levels in urine determined by the creatinine urinary assay kit (Cayman Chemicals) and expressed as percentage of the baseline concentration. Statistical analysis Values in the manuscript are means±s.e.m. For comparison of two groups, we used t -test. For more than two groups one-way analysis of variance (ANOVA) and Newman–Keuls post hoc test or two-way repeated-measures ANOVA followed by Bonferroni post hoc test were employed. On the basis of the s.d. of infarcts that we had determined in previous experiments (25% of means), we chose a sample size of 8 to 10 to detect a 40% reduction of infarct size with a power of 0.8 and an α error of 0.05 when using one-way ANOVA with four groups. How to cite this article: Rahman, M. et al. The β-hydroxybutyrate receptor HCA 2 activates a neuroprotective subset of macrophages. Nat. Commun. 5:3944 doi: 10.1038/ncomms4944 (2014).